Metal and carbene organocatalytic relay activation of alkynes for stereoselective reactions Transition metal and organic catalysts have established their own domains of excellence. It has been expected that merging the two unique domains should provide complimentary or unprecedented opportunities in converting simple raw materials to functional products. N -heterocyclic carbenes alone are excellent organocatalysts. When used with transition metals such as copper, N -heterocyclic carbenes are routinely practiced as strong-coordinating ligands. Combination of an N -heterocyclic carbene and copper therefore typically leads to deactivation of either or both of the two catalysts. Here we disclose the direct merge of copper as a metal catalyst and N -heterocyclic carbenes as an organocatalyst for relay activation of alkynes. The reaction involves copper-catalysed activation of alkynes to generate ketenimine intermediates that are subsequently activated by an N -heterocyclic carbene organocatalyst for stereoselective reactions. Each of the two catalysts (copper metal catalyst and N -heterocyclic carbene organocatalyst) accomplishes its own missions in the activation steps without quenching each other. One essential objective in chemical synthesis is to convert readily available and inexpensive starting materials to functional molecules. Transition metal catalysts are widely explored to accomplish many of these activations and chemical transformations [1] , [2] . In the last decade or so, the use of simple organic molecules as catalysts (organocatalysis) has received increasing attentions with impressive success [3] , [4] , [5] . Concurrently, it has been envisioned that merging transition metal and organocatalysts should provide a powerful strategy in chemical synthesis [6] . One of the key challenges, on the other hand, lies in the search of metal and organic catalysts that can work together cooperatively without quenching each other. In the past, organocatalysts exhibiting weak metal-coordination abilities have successfully been combined with transition metal catalysis in elegant reactions. A relatively well-studied system in this direction includes a combined use of a transition metal (such as gold, palladium, iridium, ruthenium) catalyst with chiral amine or phosphoric acid catalysts [7] , [8] , [9] , [10] , [11] , [12] , [13] , [14] . In contrast, the combined use of N -heterocyclic carbenes(NHCs) as organocatalysts [15] , [16] , [17] , [18] that can likely behave as strong-coordinating ligands [19] , [20] , [21] , [22] with transition metal catalysts remains challenging. Several efforts have been directed towards addressing such metal/organic catalysts’ quenching issues. These efforts include the use of step-by-step protocols of sequential addition of catalysts [23] , the introduction of additional coordinating ligands to compete with the organocatalysts [24] , [25] and the use of early transition metals that do not show strong-coordinating properties [26] , [27] . We are interested in combining copper [28] , [29] , [30] and NHCs for cooperative metal/organic catalysis. To the best of our knowledge, a simple combination of transition metal such as copper and strong-coordinating NHC (as organocatalyst) remains challenging and elusive [23] , [24] , [25] , [26] , [27] . Here we report the first success in using Cu and NHC cooperative catalysis for a direct activation of alkyne for stereoselective reactions ( Fig. 1a ). The reaction ( Fig. 1b ) starts with Cu-catalysed activation of alkyne to react with TsN 3 to eventually generate ketenimine [31] , [32] III as a key intermediate. This ketenimine intermediate ( III ) from the Cu-catalysed cycle is then activated by the NHC catalyst present in the same reaction solution to form azolium enamide (similar to an enolate) intermediate IV that can react with electrophilic substrates such as reactive ketones and imines to form the final product. Notably, this organocatalytic cycle also constitutes the first study in using NHC to activate ketenimine. The overall metal/organic relay catalytic processes activate readily available alkynes as enolate equivalent intermediates (azolium enamides) for stereoselective reactions. 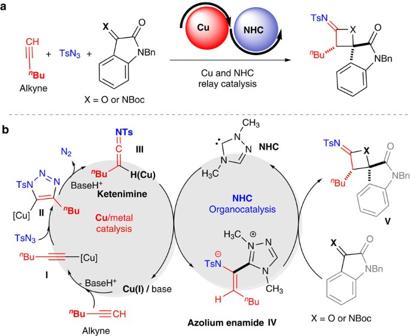Figure 1: Combined Cu and NHC cooperative relay activation of alkynes as enolate equivalents. (a) Alkyne and azide activated by Cu/NHC relay catalysis undergo formal [2+2] clycoaddition to give spiro-oxindole products. (b) Copper-catalysed [3+2] cycloaddtion of azide to alkyne gives triazoleIIthat decomposes to ketenimineIIIwith a release of N2. Addition of NHC to ketenimineIIIgives azolium enamideIV, which undergoes formal [2+2] cycloaddtion with isatin (or isatin–imine) to afford productV. NHC,N-heterocyclic carbene. Figure 1: Combined Cu and NHC cooperative relay activation of alkynes as enolate equivalents. ( a ) Alkyne and azide activated by Cu/NHC relay catalysis undergo formal [2+2] clycoaddition to give spiro-oxindole products. ( b ) Copper-catalysed [3+2] cycloaddtion of azide to alkyne gives triazole II that decomposes to ketenimine III with a release of N 2 . Addition of NHC to ketenimine III gives azolium enamide IV , which undergoes formal [2+2] cycloaddtion with isatin (or isatin–imine) to afford product V . NHC, N -heterocyclic carbene. Full size image Compatibility and reactivity of NHC and Cu catalysts We first studied the compatibility of Cu and NHC catalysts under different conditions. As summarized in Fig. 2a , while strong bases (such as NaH, KO t Bu, DBU) promote the formation of NHC-Cu complex B from the corresponding triazolium NHC pre-catalyst A and CuI, weak bases (such as TEA, DIEA, K 2 CO 3 ) led to little NHC-Cu complex after several hours. In our prior studies [27] , [33] , [34] , [35] , it is known that weak bases such as DIEA or K 2 CO 3 are sufficient for the deprotonation of triazoliums to form the carbene catalyst. We therefore concluded that under ‘weak’ base conditions, there is a controllable kinetic/thermodynamic window that allows the carbene organocatalyst and Cu metal catalyst to co-exist with a meaningful level of concentrations. In addition, we found that both the CuI and NHC-Cu complex can catalyse alkyne activation in a model reaction that converted alkyne to amide ( Fig. 2b ). This result showed that the triazolium NHC catalyst would NOT kill the ability of Cu catalyst to activate alkyne. Last, we found that NHC catalyst A could activate (pre-prepared) ketenimine substrate for nucleophilic addition to isatin 3a to form adduct 4a that was simultaneously transformed to alkene product 5a ( Fig. 2c ), suggesting that we might be able to use NHC to activate the ketenimine intermediate ( III , Fig. 1b ) generated from a Cu catalytic cycle in a relay pathway. 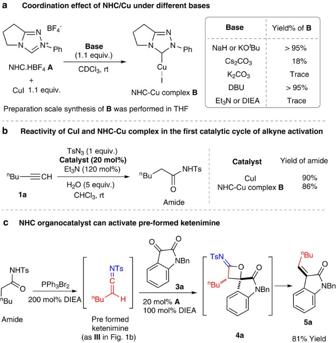Figure 2: Studies on the compatibility and reactivity of NHC and Cu catalysts. SeeSupplementary Methodsfor details. (NHC,N-heterocyclic carbene. DBU, 1,8-diazabicyclo[5.4.0]undec-7-ene, DIEA, diisopropylethylamine. Figure 2: Studies on the compatibility and reactivity of NHC and Cu catalysts. See Supplementary Methods for details. (NHC, N -heterocyclic carbene. DBU, 1,8-diazabicyclo[5.4.0]undec-7-ene, DIEA, diisopropylethylamine. Full size image Reaction optimization Encouraged by the above results ( Fig. 2 ), we moved to study the one-pot relay catalytic reactions using alkyne 1a and isatin 3a as model substrates ( Table 1 ). As expected based on our study briefed in Fig. 2 , no proposed product ( 4a or 5a ) was observed when only NHC catalyst ( A ) or the transition metal catalyst (CuI) was used ( Table 1 , entries 1–2). The isatin starting material ( 3a ) remained (entries 1–2). The use of base DIEA led to product 5a in 91% yield (entry 3). A switch of DIEA to a stronger DBU base led to a much dropped 20% yield (entry 4). This base effect is in consistence with the compatibility studies ( Fig. 2a ): strong base led to NHC-Cu complex formation and thus removed free NHC organocatalysts from the reaction mixture. Other weak bases such as K 2 CO 3 and Cs 2 CO 3 performed well (entries 5–6). An evaluation of the NHC and Cu catalyst ratios indicated that increasing the relevant amount of Cu metal catalyst has little influence of the reaction outcomes, while increasing the amount of NHC organocatalyst led to dropped product yields ( Supplementary Table 1 ). In addition, using NHC/Cu catalyst in a ratio of 1:1 (10 mol% each, entry 8) gave much better results than using the preformed NHC-Cu complex B (10 mol%). The results suggest that under the condition, the two catalysts (NHC and Cu) independently (rather than as the metal–carbene complex form) work in the relay catalysis system. Table 1 Condition optimization for Cu/NHC relay catalytic reaction. Full size table Substrate scope with isatin as electrophile substrates Under the optimized condition ( Table 1 , entry 3) the reaction was general with respects to both the alkyne and isatin substrates, as summarized in Fig. 3a . All the alkene products are characterized by 1 H, 13 C NMR and HRMS techniques ( Supplementary Figs 1–16 and Supplementary Methods ). Notably, our catalytic reaction exclusively affords Z -alkene isomer in all cases. It should be noted that such Z -alkenes are difficult to make using other approaches. For example, with Wittig reaction strategy (isatin and ylide as substrates) the use of alkyl ylides gave poor yields and poor E / Z selectivities [36] , [37] In Knoevenagel-type condensation reactions between oxindole and alkyl aldehydes, E -selective alkene products were typically obtained [38] . The radical ring closure approach for this type of products also favours E -alkenes especially for alkyl alkyne substrates [39] , [40] , [41] . In our approach, silane-protected acetylene ( 5i–5k ) can also be prepared. In a previous approach [42] such molecule could only be synthesized via radical ring closure with moderate yield and selectivity (up to 67% yield, 4.7:1 Z / E ). 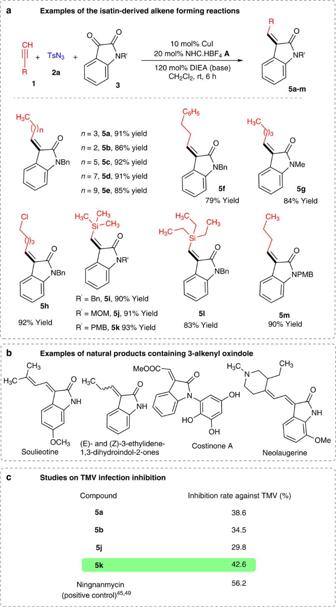Figure 3: Scope of the reaction and bio-activities of the products. Bn, benzyl; Me, methyl; MOM, methoxymethyl; PMB, para-methoxybenzyl. Figure 3: Scope of the reaction and bio-activities of the products. Bn, benzyl; Me, methyl; MOM, methoxymethyl; PMB, para-methoxybenzyl. Full size image Bio-activities of 3-alkenyl-oxindoles Our other motivation to develop methods for isatin-derived alkene products is driven by the utilities of this class of molecules. 3-Alkenyl-oxindoles is a privileged scaffold in medicinal molecules and natural products ( Fig. 3b ). For example, a novel class of receptor tyrosine kinase inhibitors synthesized from 3-alkenyl oxindole and has been used as anticancer and arthritis drugs [43] . Our laboratories are interested in plant viruses that cause detrimental effects on agriculture and horticulture [44] . One particular virus under our studies is tobacco mosaic virus (TMV). TMV is known to infect more than 400 plant species such as tobacco, tomato, potato and cucumber to cause tremendous economic loss worldwide [45] , [46] . Built on our previous studies in this area to treat plant virus diseases [47] , [48] , our preliminary studies here found that the isatin-derived alkene compound 5k showed a promising 42.6% inhibition rate against TMV infection. The positive control experiment using the commercially used drug Ningnanmycin [45] , [49] showed 56.2% inhibition rate ( Fig. 3c ). Substrate scope with isatin–imine as electrophile substrates To further demonstrate the reaction generality and expand the product diversity of our Cu/NHC metal/organic relay catalytic strategy, we evaluate the isatin-derived imine ( 6 ) as electrophile substrate ( Fig. 4a ). Initial studies using the above condition for the isatin ketone substrate ( Table 1 , entry 3) gave product 7a with a low yield (17%). Further studies (see Supplementary Table 2 ) found that by using CsF as the base, the spirocyclic β-lactam type products (spiro-azetidine oxindoles 7a–g ) were obtained as a single diastereomer (> 99:1 dr) with good yields. The use of Cs 2 CO 3 as base could also give the product, but in a slightly lower yield (see Supplementary Table 2 ). The reaction is general with respect to both alkyne and the isatin–imine substrates. All the lactam products are characterized by 1 H, 13 C NMR and HRMS techniques ( Supplementary Figs 17 and 19–30 and Supplementary Methods ). The structure and stereochemistry of a model compound 7a were unambiguously confirmed by single crystal X-ray analysis (see Supplementary Fig. 18 and Supplementary Table 3 ). Enantioselective reactions are also feasible. When chiral triazolium NHC pre-catalyst C was used, the spirocyclic lactam products (for example, 7e, 7f and 7g ) were obtained in good yields and moderate er ( Fig. 4b ). Further studies in developing highly enantioselective NHC organocatalysts for this class of reactions are under progress. 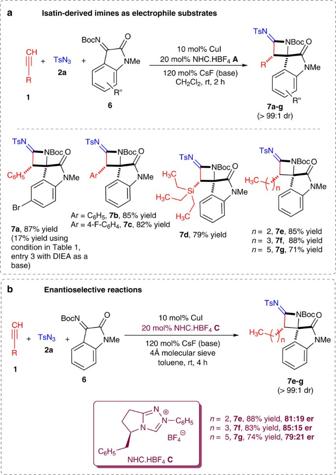Figure 4: Imines as electrophile substrates in the Cu/NHC relay catalysis system. The minor diastereomer of the product7a–gwas not detected. Figure 4: Imines as electrophile substrates in the Cu/NHC relay catalysis system. The minor diastereomer of the product 7a–g was not detected. Full size image In summary, we have developed a cooperative relay catalysis strategy using NHCs as organocatalysts and Cu as a transition metal catalyst. Under a properly chosen condition (such as the use of weak base to modulate the formation of free carbene and NHC-Cu complex), Cu metal catalyst and triazolium NHC organic catalyst work independently to accomplish its own mission without quenching each other. Our overall one-pot multistep reaction, consisting of the first NHC organocatalytic activation of ketenimine, converts readily available alkynes as enamide intermediates for stereoselective reactions. This study suggests that by properly controlling the kinetics and/or thermodynamics of metal/organic catalyst coordination, organic catalysts and tradition metals that were typically considered to form strong metal–organic coordination can likely be combined for cooperative catalysis. Encouraged by the present results, our next step is to develop general strategies for metal/organic cooperative catalysis that can work for a broad set of catalyst systems for new activations and reactions. Materials For 1 H, 13 C NMR and HPLC spectra of compounds in this manuscript, see Supplementary Figs 1–30 . For details of the synthetic procedures, see Supplementary Methods . Synthesis of 5a A dry 10-ml Schlenk tube equipped with a magnetic stirring bar was successively charged with 1 -hexane 1a (44.1 μl, d =0.723 g ml −1 , 31.9 mg, 0.39 mmol), tosyl azide 2a (70.9 mg, 0.36 mmol), N -benzyl isatin 3a (71.1 mg, 0.30 mmol) and CuI (5.6 mg, 0.03 mmol) and NHC pre-catalyst A (16.4 mg, 0.06 mmol). The tube was closed with a septum, evacuated and refilled with nitrogen. To this mixture was added dry dichloromethane (1.0 ml), followed by the addition of DIEA (62.5 μl, d =0.742 g ml −1 , 46.4 mg, 0.36 mmol) via a microsyringe. After stirring for 6 h at room temperature, the reaction mixture was concentrated under reduced pressure. The crude residue was directly applied to silica gel column chromatography (hexanes/ethyl acetate) to afford Z )-1-benzyl-3-pentylideneindolin-2-one ( 5a, 79.5 mg, 91% yield). Synthesis of 7a A dry 10-ml Schlenk tube equipped with a magnetic stirring bar was successively charged with phenyl acetylene (42.7 μl, d =0.930 g ml −1 , 39.7 mg, 0.39 mmol), tosyl azide 2a (0.36 mmol), isatin-derived imine 6 (101.4 mg, 0.30 mmol), CuI (5.6 mg, 0.03 mmol) and NHC pre-catalyst A (16.4 mg, 0.06 mmol). The tube was closed with a septum, evacuated and refilled with nitrogen. To this mixture was added dry dichloromethane (1.0 ml), followed by the addition of CsF (54.3 mg, 0.36 mmol). After stirring for 2 h at room temperature, the reaction mixture was concentrated under reduced pressure. The crude residue was directly applied to silica gel column chromatography (hexanes/ethyl acetate) to afford tert -butyl ( E )-5′-bromo-1′-methyl-2′-oxo-3-phenyl-4-(tosylimino)spiro[azetidine-2,3′-indoline]-1-carboxylate ( 7a, 182.7 mg, 87% yield). Accession codes: The X-ray crystallographic coordinates for structures reported in this Article have been deposited at the Cambridge Crystallographic Data Centre (CCDC), under deposition number CCDC 981345. These data can be obtained free of charge from The Cambridge Crystallographic Data Centre via www.ccdc.cam.ac.uk/data_request/cif . How to cite this article: Namitharan, K. et al. Metal and carbene organocatalytic relay activation of alkynes for stereoselective reactions. Nat. Commun. 5:3982 doi: 10.1038/ncomms4982 (2014).